Acoustic dynamics of network-forming glasses at mesoscopic wavelengths The lack of long-range structural order in amorphous solids induces well known thermodynamic anomalies, which are the manifestation of distinct peculiarities in the vibrational spectrum. Although the impact of such anomalies vanishes in the long wavelength, elastic continuum limit, it dominates at length scales comparable to interatomic distances, implying an intermediate transition regime still poorly understood. Here we report a study of such mesoscopic domains by means of a broadband version of picosecond photo-acoustics, developed to coherently generate and detect hypersonic sound waves in the sub-THz region with unprecedented sampling efficiency. We identify a temperature-dependent fractal v 3/2 frequency behaviour of the sound attenuation, pointing to the presence of marginally stable regions and a transition between the two above mentioned limits. The essential features of this behaviour are captured by a theoretical approach based on random spatial variation of the shear modulus, including anharmonic interactions. Vibrational states of glasses in the low-frequency regime are often described in terms of quantized plane-wave phonon modes, resembling those of the crystalline counterpart. On the other hand, the amorphous state induces a number of peculiar low-temperature properties regardless of the specific structure of the material, from covalently bound glasses to polymers and biological matter. These properties include anomalous acoustic behaviour, the existence of a plateau in the temperature ( T ) dependence of the thermal conductivity, the peak in the T dependence of C p / T 3 (where C p is heat capacity at constant pressure) and the ‘boson peak’ observed in inelastic scattering of light or neutrons at meV energies, that is, an excess of vibrational density of states g ( v ) over the prediction of the Debye model, expressed as g ( v )/ v 2 (typical energy scale: a few millielectronvolts) [1] , [2] . There is a consensus that the boson peak is a manifestation of some sort of disorder, and it is believed to be key to fundamental understanding of the vibrational states of glassy and amorphous materials, which are beyond the simple plane-wave phonon picture for crystals. Nevertheless, its physical origin has remained a serious puzzle in condensed-matter physics and materials science. Among the disorder-sensitive properties, the frequency dependence of the sound attenuation coefficient ( Г ), in particular, appears to be the result of an interplay of several physical mechanisms from the ultrasonic to the THz frequency regimes [3] , [4] , [5] , [6] , [7] , [8] , [9] , [10] , [11] , [12] , [13] , [14] . On a qualitative ground, one would expect that—in the very long acoustic wavelength limit—the effect of disorder vanishes out and a crystal-like picture holds (except for the fact that long-wavelength longitudinal waves of a glass are attenuated). In fact, such a behaviour is observed up to few tens of GHz in ultrasonics (US) and Brillouin light scattering (BLS) experiments [8] . In the low-frequency regime (MHz to GHz regime, acoustic wavelength λ a >100 nm), where the wave picture holds, the sound attenuation is expected to be governed by internal friction due to anharmonic interactions like in dielectric crystals. Therefore, the classical theory of sound attenuation in crystals, founded by Landau and Akhiezer [4] , [6] , [15] , [16] has been used also for glasses [8] , [10] , [11] . These theories [6] predict a v 2 law, which should saturate at some characteristic frequency, and a direct proportionality with T . In fact, the v 2 behaviour has been observed up to few tens of GHz in US and BLS experiments [8] . Several models for the influence of relaxation processes on sound attenuation in glasses have been considered [5] , [7] , [9] , [17] . In the opposite limit, when the dominant acoustic wavelength approaches the average inter-particle distance, the structural disorder becomes of crucial importance. The corresponding frequency region (THz) is accessible by inelastic neutron scattering (INS) and inelastic X-ray scattering (IXS) experiments [18] and by molecular dynamics(MD) simulations. Experiments indicate also here a v 2 but temperature-independent behaviour of the sound attenuation, albeit with a different (higher) coefficient. Hence, consist with recent observations at the edge of the IXS accessible window [19] , [20] , one legitimately expects a crossover between these two regimes, which should occur at frequencies between 50 GHz and 1 THz, ruled by a v 4 behaviour, which is expected for elastic scattering in a statically disordered medium (Rayleigh scattering [3] ). In this work, we investigate the propagation of hypersonic waves in the mesoscopic domain in between the two regimes by means of a newly developed broadband version of picosecond photo-acoustics (BPA), a technique that we recently introduced [21] building on a 1 kHz regeneratively amplified Ti:Sa laser system. Specifically, we report experimental data for sound attenuation in the prototypical strong-glass vitreous germania (v-GeO 2 ), obtained by low-pressure chemical vapour deposition (LPCVD), accessing the ≈100 GHz frequency gap existing between BLS and IXS. We find a temperature-dependent, fractal frequency behaviour of the acoustic attenuation, signalling the presence of marginally stable regions and anticipating the transition to the disordered dominated regime, occurring in the boson peak region. A theoretical approach based on random spatial variation of the shear modulus including anharmonic interactions accounts for the observed features. Identification of the Rayleigh crossover Experimental values of Г( v ), obtained in v-GeO 2 with different techniques (US (refs 22 , 23 ), BLS (refs 24 , 25 , 26 ), INS (ref. 24 ) experiments and MD (ref. 24 ) simulations) are compared with the present experimental results in Fig. 1 . 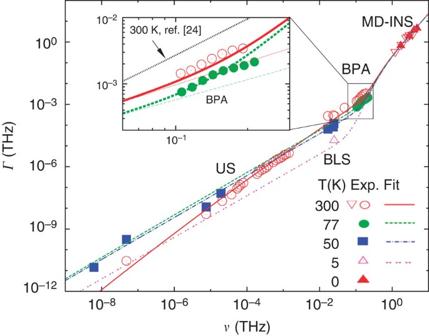Figure 1: Acoustic attenuation in GeO2over 10 frequency decades. Г(v) obtained by different techniques at different temperatures, along with the best fit with equations 1, 2, 3, as indicated in the table. Belowv=1 THz a strong temperature dependence is observed, a clear signature of anharmonicity. The Broadband picosecond photo-acoustics (BPA) data are the result of an interpolation of 1340 different wavelengths, corresponding to each single channel of optical multichannel analyser. The inset magnifies the BPA data, error bars are smaller that the symbol size. A significant departure from the purely anharmonic contribution (thin lines in the inset) is clearly observed for both temperatures. The thin black dotted line is the best fit before BPA data atT=300 K condition24. Best fitting parameters areτ0=1.45 × 10−4ps,σV=2469 K,vc=0.443 THz,A=0.1313 andB=0.233 ps. Figure 1: Acoustic attenuation in GeO 2 over 10 frequency decades. Г ( v ) obtained by different techniques at different temperatures, along with the best fit with equations 1, 2, 3, as indicated in the table. Below v =1 THz a strong temperature dependence is observed, a clear signature of anharmonicity. The Broadband picosecond photo-acoustics (BPA) data are the result of an interpolation of 1340 different wavelengths, corresponding to each single channel of optical multichannel analyser. The inset magnifies the BPA data, error bars are smaller that the symbol size. A significant departure from the purely anharmonic contribution (thin lines in the inset) is clearly observed for both temperatures. The thin black dotted line is the best fit before BPA data at T =300 K condition [24] . Best fitting parameters are τ 0 =1.45 × 10 −4 ps, σ V =2469 K, v c =0.443 THz, A =0.1313 and B =0.233 ps. Full size image In order to identify the crossover frequency between the low/high-frequency regimes, we first make use of a fitting model, used in the previous literature, combining additively an anharmonic and a disorder scattering contribution [24] , [27] . As the data below ≈100 GHz cannot be described with a simple Akhiezer-like v 2 behaviour (they show a linear dependence upon approaching the crossover region from below), we used an anharmonic contribution ( Г Th ) allowing for a spatially varying relaxation time τ ( V ) with a half-gaussian distribution of activation parameters V (the so called TARP scheme [7] , thermally activated relaxation processes, see Supplementary Note 1 for further details). the Г Th contribution follows a v 1 law in the frequency range corresponding to the relaxation rate distribution, as showed in Supplementary Fig. S1 . The scattering contribution Г sc just interpolates between a Rayleigh v 4 to a high-frequency v 2 law with crossover v c , which should be below (but near to) the boson peak frequency v B [12] , [28] . Equations 1, 2, 3 was previously applied to estimate v c [24] obtaining a value of ≈60 GHz, that is, one order of magnitude below the boson peak located at v B ~750 GHz (ref. 29 ). Our new BPA measurement for two different temperatures unambiguously indicates a significant up-shift of v c to ~450 GHz, which is much closer to v B . Remarkably, the temperature dependence of our BPA data, as shown in the inset of Fig. 1 , still indicates a strong anharmonic contribution in the 100 GHz region. Theoretical description of the crossover region In order to describe the crossover region accounting for the observed anharmonic behaviour, we now introduce a theoretical description, building on an inhomogeneous version of elasticity theory [30] in which the local shear modulus is assumed to fluctuate in space (heterogeneous elasticity theory [12] , [14] , [28] , [31] ) with a Gaussian distribution. The theory, outlined in Methods section, depends on a single parameter γ —the fluctuation of the elastic constants—which is a measure of the disorder of the system, upper limited by a critical value γ c , which sets an instability threshold. It allows determining the dynamic susceptibility by means of self-consistent equations involving a self-energy Σ. The acoustic attenuation Г relates to the imaginary part of the self-energy via: Г( v ) v Σ′′( v ). Away from the instability, for γ < γ c , the self-energy can be conveniently evaluated within the harmonic approximation giving rise to the temperature-independent contribution Σ har ( v ), solely dependent on the system disorder γ . The harmonic approximation captures important experimentally observed features related to the boson peak: it reconciles the Brillouin (GHz) and the IXS (THz) regimes via a Г v 4 to a Г v 2 crossover. It does not explain, however, the significant temperature dependence observed in our BPA data in the 100 GHz regime and below. A way to account for such experimentally observed temperature dependence is to introduce the lowest order linear correction in T to the harmonic self-energy into the self-consistent equations. Right at the instability the combined presence of anharmonicity and disorder causes a fractal frequency dependence of the sound attenuation as well as the density of vibrational states Г ( v ) T 1/2 v 3/2 and g ( v ) v 3/2 , away from the instability the harmonic approximation is retrieved. A satisfactory description of our data, including the presence of the crossover and the sub-THz temperature dependence is therefore obtained by an incoherent superposition of sub critical and critical self energies: The prediction of the theory is shown in Fig. 2 , against the available sound attenuation data on GeO 2 above 100 GHz. A good description is obtained with γ c − γ =0.01 and x =0.144 ( T =77 K) or x =0.146 ( T =300 K). As can be observed, the transition to the upper v 2 range is consistent with the crossover frequency v c ~450 GHz obtained in the phenomenological fit of Fig. 1 , and the experimental Г v ( vT ) 1/2 temperature dependence of sound attenuation is correctly reproduced. 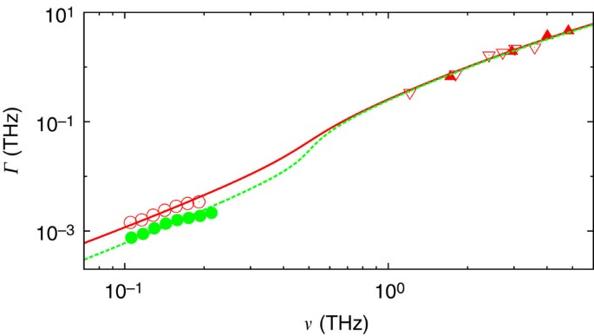Figure 2: Acoustic attenuation in GeO2. Description of the crossover region based on heterogeneous elasticity theory (T=300 K solid line,T=77 K dashed line). Experimental data are the same as inFig. 1. Figure 2: Acoustic attenuation in GeO 2 . Description of the crossover region based on heterogeneous elasticity theory ( T =300 K solid line, T =77 K dashed line). Experimental data are the same as in Fig. 1 . Full size image We presented experimental data for hypersonic attenuation in a strong glass obtained in a previously unexplored frequency region, suggestive of the presence of a crossover from continuous wave to coarse grained elasticity occurring just below the boson peak. The crossover, located around 450 GHz, corresponds to an acoustic wavelength of nm, representing the correlation length associated with the transition. This lengthscale, in turn, comprises ≈25 GeO 4 tetrahedral units [32] . Let us now discuss on the similarities and differences of the sound attenuation in the two network glasses GeO 2 and SiO 2 . At high frequencies, (THz region)–as evidenced by IXS, neutron and simulation data–the sound attenuation varies as v 2 above the boson peak frequency, which is situated at ~1.2 THz in SiO 2 (ref. 20 ) and ~0.75 THz in GeO 2 (ref. 29 ). In SiO 2 , the sound attenuation below the boson peak frequency drops with a stronger frequency dependence indicating the onset of a Rayleigh law [20] . In GeO 2 , the corresponding frequency window lies outside the IXS accessible range. At very low frequencies, where anharmonic relaxation processes dominate, the attenuation SiO 2 shows an Akhiezer-like v 2 dependence (that is, driven by a single relaxation time) holding up to frequencies as high as 600 GHz (refs 33 , 34 ), whereas in GeO 2 a v 1 law is observed, indicating a similar mechanism but with a broad distribution of relaxation times. A self-consistent theory based on spatial fluctuation of shear moduli—including anharmonic interactions—is here presented to account for the temperature-dependent damping in the crossover region. This is achieved advancing the idea of marginally stable regions ( γ = γ c ), surrounded by a ‘host’ with γ < γ c . Marginally stable regions have been detected in computer simulations of a metallic glass [35] and in model glasses [36] . More recently, simulations of a soft-sphere glass [31] show, in fact, that both the frequency-fractal behaviour and a boson peak are present in agreement with the present experimental result. The former are also responsible for the fractal frequency dependence of vibrational density of states g ( ω ) ω 3/2 , while the latter explains the dip in the frequency dependent sound velocities occurring at the crossover [12] , [28] , [31] . Our work unambiguously demonstrates that marginally stable regions exist in a real glass, and we anticipate that this might be a general feature of the amorphous state. We note that the slight increase of the concentration of marginally stable regions with temperature, linearly extrapolated towards the glass transition ( T g =980 K) would lead to a critical concentration of about x c ≈15%. This value, however, should be taken as a lower bound, because we expect a steeper temperature dependence upon approaching T g . It has been advanced in the recent literature that marginally stable regions are directly related to shear transformation zones in metallic [35] , [37] and model [38] glasses. Our result demonstrates the existence of these regions in network-forming glasses, providing a way to estimate the critical density [39] by performing BPA experiments close to T g . Broadband picosecond acoustics A schematic layout of the BPA setup is shown in Fig. 3 . It is based on a regeneratively amplified Ti:sapphire laser producing 50 fs, 4 mJ pulses at 800 nm wavelength and 1 kHz repetition rate. A portion of the beam (the pump, with energy up to 5 μJ), after passing through a delay line, is loosely focused on the sample. A thin metallic coating launches by ‘instantaneous’ thermal expansion a longitudinal acoustic wavepacket with a characteristic spectrum extending in the 40–400 GHz region [40] . The acoustic pulse then travels inside the sample and its motion is probed by a second delayed optical pulse. 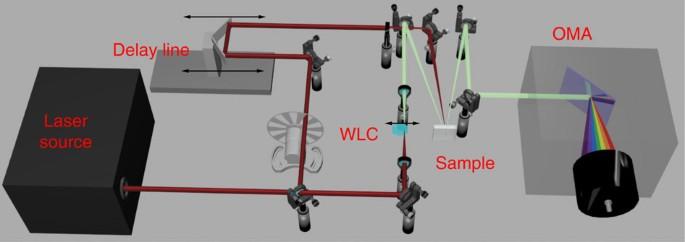Figure 3: Schematics of the pump-probe setup. A small fraction of the Ti:sapphire pulsed source acts as pump, while the broadband probe (optically delayed with respect to the pump) is obtained through generation of WLC in CaF2. The probe, after the interaction with the sample, is analysed by an optical multichannel analyser. Figure 3: Schematics of the pump-probe setup. A small fraction of the Ti:sapphire pulsed source acts as pump, while the broadband probe (optically delayed with respect to the pump) is obtained through generation of WLC in CaF 2 . The probe, after the interaction with the sample, is analysed by an optical multichannel analyser. Full size image In our realization of the experiment, outlined in Fig. 3 , the probe is a broadband pulse obtained by focusing a fraction of the laser light onto a 2-mm thick CaF 2 plate to generate a stable broadband single-filament white light continuum (WLC). After the interaction with the sample, a visible portion of the WLC, extending from 380 to 650 nm, is dispersed on an optical multichannel analyser [21] . Impinging on the sample, each wavelength ( λ pr ) in the probe pulse is reflected by the acoustic strain wave through a (stimulated) Brillouin scattering process, that is, interacts with a single phonon of frequency where c L is the (longitudinal) sound velocity, q the modulus of the phonon wavevector (equal to the exchanged light momentum), n ( λ pr ) the refractive index of the medium and θ the scattering angle. The Brillouin scattered intensity interferes with the portion of probe beam reflected by the fixed metallic layer, leading to time-dependent oscillations reported in Fig. 4 as the relative (with and without the pump pulse) variation of transient reflectivity for different time delays ( ). The periodicity and damping of such oscillations, set by the Bragg condition and corresponding to the period of the phase-matched acoustic phonon [41] , gives direct access to acoustic parameters such as sound velocity and attenuation in the same frequency range as BLS experiments. 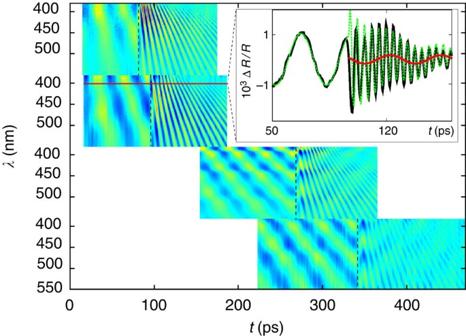Figure 4: Broadband picosecond acoustics data. Colour map of pump-probe signal (after the subtraction of thermal background) atT=77 K for different GeO2thicknesses (from left to right 302-370-1020-1320, nm). A strong damping effect of fast oscillations at the silicon interface upon increasing thickness can be observed. The inset shows a single wavelength temporal trace (black thick line), and its best fit (green dashed line) with the three components representing the acoustic wave launched in the sample, transmitted and reflected at the silicon interface. This latter, relatively small contribution is shown by the red line. Figure 4: Broadband picosecond acoustics data. Colour map of pump-probe signal (after the subtraction of thermal background) at T =77 K for different GeO 2 thicknesses (from left to right 302-370-1020-1320, nm). A strong damping effect of fast oscillations at the silicon interface upon increasing thickness can be observed. The inset shows a single wavelength temporal trace (black thick line), and its best fit (green dashed line) with the three components representing the acoustic wave launched in the sample, transmitted and reflected at the silicon interface. This latter, relatively small contribution is shown by the red line. Full size image Critically, as shown in Devos et al . [42] the presence of a silicon substrate, in a metal/sample/Si structure, allows extending upwards the accessible acoustic frequency range as, when entering the Si substrate, the phase-matched acoustic frequency is enhanced by the larger value of sound speed ( 8430, m s −1 ) and refractive index ( at λ pr =372 nm) compared with germania ( m s −1 , n (GeO2) ~1.65). Consequently, by probing the acoustic wave at the sample/substrate interface, the accessible frequency region can be upscaled to the 100 GHz decade, a range of paramount importance in amorphous materials science, showing an extremely rich phenomenology. A set of samples of different thicknesses (302-370-1020-1320, nm) was obtained by a single LPCVD on the polished surface of a [100] silicon wafer (see Supplementary Methods ). An equal thickness (10 nm) of Ti transducer layer was deposited on top all samples to ensure identical acoustic wavepacket properties for the whole series. Transient reflectivity data, , are first reduced by subtraction of a thermal background [43] , as performed in Devos et al . [42] . The results are shown in Fig. 4 : sinusoidal best fits of for each wavelength and each GeO 2 thickness [21] (see an example in the inset in Fig. 4 ), bears information on the intensity of the acoustic wave travelling in GeO 2 first and then in the Si substrate. The evolution of the oscillation amplitude at the interface GeO 2 /Si ( A si ) for different sample thicknesses L , (normalized to the amplitude in the GeO 2 , , to account for possible sample dependent variations of the induced acoustic wavepacket) is a measure of the acoustic damping in the sample α ac ( v ), and reads: Following the procedure proposed in Refs 44 , the factor f , depending on the thickness and optical properties of the different sample layers, was used to keep into account for multiple reflection effects. The α ac ( v ) relates to the acoustic energy mean free path via l −1 =2 α ac ( v ). In terms of the acoustic damping measured in the frequency domain Г ( v ) (full-width at half maximum of Brillouin line) we have Measurements were performed at both room and liquid nitrogen temperatures [44] . Generalized elasticity theory As outlined in Results section, the theory that we present is an inhomogeneous version of elasticity theory, where the shear modulus is assumed to fluctuate in space [12] , [14] , [28] , [31] with a Gaussian distribution with corresponding average G 0 and variance . The disorder-induced fluctuations cause a frequency dependence in the macroscopic shear and longitudinal moduli where ω =2π v is the angular frequency and c L,T ( ω ) are the (complex) longitudinal and transverse sound velocities, ρ is the mass density, and Σ( ω ) is the complex self-energy function. The c L,T ( ω ) fluctuations rule the longitudinal and transverse susceptibilities: If the local bulk modulus K is assumed not to fluctuate in space, then its macroscopic counterpart is frequency independent, and we have The acoustic wave attenuation is related to the imaginary part of the self-energy by the relation Г( ω ) ω Σ′′( ω ). The purely disorder-induced frequency dependence of the attenuation can be described by the harmonic self-energy function Σ harm ( ω ). where is the dimensionless disorder parameter. By solving the self-consistent equation 7 to equation 10, we obtain the solution for Σ harm ( ω ) within the so called self-consistent Born approximation (SCBA). Let us now introduce anharmonicity. This can be achieved by including the non-linear terms of standard elasticity theory [30] into the Lagrangian of the theory [14] . The result is–to the lowest order in the anharmonicity—a self-energy whose imaginary part varies linearly with frequency and temperature like in Akhiezer’s theory for the transverse sound attenuation of crystals [4] . It had been noted already some time ago [45] that the combined effect of the anharmonicity and disorder in the vicinity of the instability can lead to a mode-coupling scaling scenario [46] with a frequency dependence Г ( ω ) ω 3/2 . Such a frequency dependence, indeed, is obtained right at the instability γ = γ c if Σ harm in the equation 10 for the dynamic susceptibilities is replaced by where A describes the strength of the anharmonicity. By solving again the self-consistent equation 7 to equation 10, one obtains the anharmonic solution for the self-energy which, in the γ ≈ γ c limit, can be written as Here B and C are (positive) coefficients relating to the harmonic theory [12] , [28] , [31] and Σ c (0) is the critical self-energy at ω =0. At marginal stability ( γ = γ c ) the anharmonic term is dominant, giving an ( ωT ) 1/2 law for Σ′′( ω ). For γ < γ c the other contributions, which describe the increase of the sound attenuation near the BP become important and the fractal law is less pronounced. An appropriate form for the self-energy [31] is the incoherent superposition of critical (frequency fractal) and sub critical contributions, according to equation 4. An important feature of the frequency-fractal contribution is that it varies with temperature as T 1/2 (see equation 12), as experimentally observed. How to cite this article: Ferrante, C. et al . Acoustic dynamics of network-forming glasses at mesoscopic wavelengths. Nat. Commun. 4:1793 doi: 10.1038/ncomms2826 (2013).